Circadian control of bile acid synthesis by a KLF15-Fgf15axis Circadian control of nutrient availability is critical to efficiently meet the energetic demands of an organism. Production of bile acids (BAs), which facilitate digestion and absorption of nutrients, is a major regulator of this process. Here we identify a KLF15- Fgf15 signalling axis that regulates circadian BA production. Systemic Klf15 deficiency disrupted circadian expression of key BA synthetic enzymes, tissue BA levels and triglyceride/cholesterol absorption. Studies in liver-specific Klf15 -knockout mice suggested a non-hepatic basis for regulation of BA production. Ileal Fgf15 is a potent inhibitor of BA synthesis. Using a combination of biochemical, molecular and functional assays (including ileectomy and bile duct catheterization), we identify KLF15 as the first endogenous negative regulator of circadian Fgf15 expression. Elucidation of this novel pathway controlling circadian BA production has important implications for physiologic control of nutrient availability and metabolic homeostasis. Bile acids (BAs) are derived from enzymatic oxidation of cholesterol and function as detergents that facilitate digestion and absorption of nutrients [1] , [2] . In addition, there is growing appreciation that BA can function as hormones to regulate systemic metabolic homeostasis [3] . Previous studies have demonstrated that BA production exhibits a distinct daily rhythm [4] , [5] , [6] , [7] but our understanding of endogenous mechanisms that regulate this process are incompletely understood. Primary BA are synthesized in the liver, stored temporarily in the gallbladder (GB), secreted into the intestine on food ingestion (to facilitate absorption of dietary lipids and fat-soluble vitamins) and then reabsorbed in the distal ileum. In addition, non-hepatic sources of BAs such as microbiota can affect BA composition and pools [8] . With respect to hepatic BA production, the major and rate-limiting enzyme in BA production is cholesterol 7α-hydroxylase ( Cyp7a1) , with minor contributions from additional enzymes such as 25-hydroxycholesterol 7α-hydroxylase ( Cyp7b1 ) [2] . Importantly, reabsorption of BAs in the distal ileum is critical as part of a negative feedback loop that inhibits BA synthesis in the liver by repressing Cyp7a1 . Studies over the past decade have revealed that feedback inhibition of BA synthesis involves ileal farnesoid X receptor (FXR/NR1H4)-induced fibroblast growth factor 15 ( Fgf15 ) [9] and hepatic FXR-induced atypical nuclear receptor small heterodimer partner ( Shp/Nr0b2 ) [10] . These studies indicate that expression of Fgf15 , which occurs principally in enterocytes of the ileum [11] , [12] , is induced by BA-mediated activation of the nuclear receptor FXR in enterocytes. FGF15 is subsequently secreted into the circulation where it is transported to the liver and binds its cognate receptor fibroblast growth factor receptor 4/FGFR4 and co-receptor βKlotho on hepatocytes [13] and activates a signalling pathway that culminates in repression of Cyp7a1 . Efforts to understand the circadian basis for BA synthesis have focused on CYP7A1 as this key enzyme exhibits robust circadian expression and activity during a day–night cycle. Several circadian transcription factors have been identified as direct transcriptional regulators of Cyp7a1 messenger RNA (mRNA) expression in hepatocytes [4] , [5] . Although several recent reports have documented that Fgf15/19 levels exhibit diurnal variation [14] , [15] , the molecular basis and functional importance in regulating circadian BA production is unknown. KLF15 regulates BA synthesis Recent work has identified the transcription factor Kruppel-like factor 15 (KLF15), as critical for nutrient flux and utilization in the context of daily feed–fast cycles [16] . Unbiased transcriptome analysis of mouse livers from wild-type ( Klf15 +/+ ) and Klf15 systemic knockout mice ( Klf15 −/− ) revealed reduced expression of Cyp7a1 and Cyp7b1 (ref. 17 ). To confirm these findings, liver tissues were harvested from control and systemic Klf15 −/− mice at 4-h intervals across a 24-h cycle (ZT0: 06:00, lights on; ZT12: 18:00, lights off). As expected, Klf15 and several BA synthetic enzymes exhibited an oscillatory expression pattern ( Fig. 1a,b ). Importantly, the oscillation of Cyp7a1 and Cyp7b1 mRNA and protein were attenuated in Klf15 −/− livers with minimal effect on sterol 27-hydroxylase ( Cyp27a1 ; Fig.1a ). Consistent with this reduction in Cyp7a1 , tissue BA levels as well as GB weight were reduced in Klf15 −/− mice ( Fig. 1c,d ). No effect was found on mRNA expression of key factors known to regulate Cyp7a1 ( Supplementary Fig. 1 ). As BAs are critical for lipid absorption, we assessed the effect of Klf15 deficiency on triglyceride (TG) and cholesterol absorption. Labelled TG and cholesterol were infused into the gut and luminal amounts assessed 6 h after infusion. Klf15 −/− mice exhibited higher levels of luminal lipids (both TG and cholesterol) in the duodenum, one of the main regions of the gastrointestinal tract involved in absorbing lipid-soluble nutrients ( Fig. 1e ). The presence of higher amount of TG or cholesterol in the duodenal lumen indicated reduced absorption, a finding consistent with the observation that BAs are decreased in the Klf15 −/− animals ( Fig. 1c ). Collectively, these findings identify KLF15 as an essential regulator for circadian expression of key BA synthetic enzymes, BA pools and fat absorption. 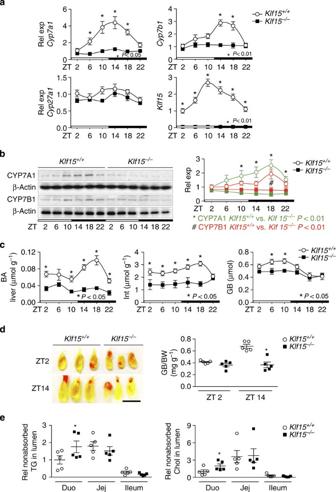Figure 1:Klf15deficiency attenuates circadian bile acid (BA) synthesis and lipid absorption. (a) The circadian mRNA relative expression (Rel Exp) of BA synthetic enzymesCyp7a1,Cyp7b1andCyp27a1as well asKlf15in wild-type (Klf15+/+) and knockout (Klf15−/−) mouse livers (five per time point).Cyp7a1,Cyp7b1andKlf15mRNA expressions exhibit endogenous circadian rhythms inKlf15+/+mouse livers (P<0.01) but the rhythms inKlf15−/−livers were lost with reduced expression at indicated time points. ZT, zeitgeber time (h). (b) Immunoblot (left) and quantification (right) of CYP7A1 and CYP7B1 protein expressions in mouse livers (representative of three experiments). The Rel Exps of CYP7A1 and CYP7B1 proteins (right) exhibit diurnal rhythm inKlf15+/+mouse livers (P<0.05) but the rhythms inKlf15−/−livers were lost with reduced expression at indicated time points. (c) BA amount in liver, intestine (Int) and gallbladder (GB) monitored in a circadian fashion (n=5). Liver and intestine BAs amount were normalized to tissue mass. The tissue BA fractions exhibit diurnal rhythm inKlf15+/+mice (P<0.01) but not inKlf15−/−mice with reduced BA amount at indicated time points. (d) GB sizes and weights normalized to body weights at ZT2 or ZT14 (n=5). Scale bar, 5 mm. (e) Triglyceride (TG) and cholesterol (Chol) absorption in small intestine. Relative amount of non-absorbed TG and Chol in three small intestinal segments: duodenum (Duo), jejunum (Jej) and ileum (n=5). Data represent mean±s.e.m. Statistical significance of circadian rhythm for each genotype was analysed using analysis of variance (one way within genotype; two way between genotypes) followed by Bonferroni post-test. Statistical significance between the two individual groups was assessed using Student’st-test. Normal distribution was assumed for all experimental groups. * and # indicateP<0.05 or 0.01, compared withKlf15+/+mice at indicated time points or relative (Rel) non-absorbed TG or cholesterol detected inKlf15+/+mouse duodenum. Figure 1: Klf15 deficiency attenuates circadian bile acid (BA) synthesis and lipid absorption. ( a ) The circadian mRNA relative expression (Rel Exp) of BA synthetic enzymes Cyp7a1 , Cyp7b1 and Cyp27a1 as well as Klf15 in wild-type ( Klf15 +/+ ) and knockout ( Klf15 −/− ) mouse livers (five per time point). Cyp7a1 , Cyp7b1 and Klf15 mRNA expressions exhibit endogenous circadian rhythms in Klf15 +/+ mouse livers ( P <0.01) but the rhythms in Klf15 −/− livers were lost with reduced expression at indicated time points. ZT, zeitgeber time (h). ( b ) Immunoblot (left) and quantification (right) of CYP7A1 and CYP7B1 protein expressions in mouse livers (representative of three experiments). The Rel Exps of CYP7A1 and CYP7B1 proteins (right) exhibit diurnal rhythm in Klf15 +/+ mouse livers ( P <0.05) but the rhythms in Klf15 −/− livers were lost with reduced expression at indicated time points. ( c ) BA amount in liver, intestine (Int) and gallbladder (GB) monitored in a circadian fashion ( n =5). Liver and intestine BAs amount were normalized to tissue mass. The tissue BA fractions exhibit diurnal rhythm in Klf15 +/+ mice ( P <0.01) but not in Klf15 −/− mice with reduced BA amount at indicated time points. ( d ) GB sizes and weights normalized to body weights at ZT2 or ZT14 ( n =5). Scale bar, 5 mm. ( e ) Triglyceride (TG) and cholesterol (Chol) absorption in small intestine. Relative amount of non-absorbed TG and Chol in three small intestinal segments: duodenum (Duo), jejunum (Jej) and ileum ( n =5). Data represent mean±s.e.m. Statistical significance of circadian rhythm for each genotype was analysed using analysis of variance (one way within genotype; two way between genotypes) followed by Bonferroni post-test. Statistical significance between the two individual groups was assessed using Student’s t -test. Normal distribution was assumed for all experimental groups. * and # indicate P <0.05 or 0.01, compared with Klf15 +/+ mice at indicated time points or relative (Rel) non-absorbed TG or cholesterol detected in Klf15 +/+ mouse duodenum. Full size image As both Klf15 and Cyp7a1 are robustly expressed in the liver, we hypothesized that hepatic KLF15 likely regulated Cyp7a1 at the transcriptional level. However, co-transfection studies failed to show any effect of KLF15 on Cyp7a1 - luciferase reporter activity at baseline or in combination with several known positive regulators of Cyp7a1 ( Supplementary Fig. 2a–d ). Further, viral overexpression or knockdown of Klf15 in hepatocytes had only a modest effect on Cyp7a1 expression ( Supplementary Fig. 2e,f ). To definitively determine whether hepatic KLF15 regulates Cyp7a1 and BA synthesis, we generated liver-specific Klf15 -knockout mice (Li-KO; Klf15 f/f ; Albumin-Cre ( Alb-Cre )). Efficient deletion of Klf15 was confirmed at both the mRNA and protein levels ( Supplementary Fig. 3a,b ). Consistent with our in vitro studies, Li-KO mice demonstrated only a minimal alteration in Cyp7a1 mRNA expression and BA pools in the tissues ( Supplementary Fig. 3c,d ). By contrast, oscillation of the minor BA regulatory enzyme Cyp7b1 was modestly reduced ( Supplementary Fig. 3c , right panel). These findings suggest a non-hepatic basis for KLF15 regulation of Cyp7a1 expression and BA synthesis. Ileal KLF15 inhibits Fgf15 An essential, non-hepatic mechanism regulating Cyp7a1 expression and BA synthesis involves ileum-derived FGF15. Previous studies show that Fgf15 is expressed in the epithelial cells of the ileum [9] but the cellular expression of Klf15 in the ileum is unknown. In situ hybridization (ISH) studies show that both Fgf15 and Klf15 mRNA are expressed in the epithelial cells of ileal villi ( Fig. 2a ; Supplementary Fig. 4a ). Overexpression of Klf15 in primary mouse small intestinal epithelial cells potently repressed, while knockdown induced, Fgf15 expression at baseline or following induction of Fgf15 by FXR agonist GW4064 ( Fig. 2b ; Supplementary Fig. 4b–d ). Gene reporter assays revealed that KLF15 repressed the Fgf15 promoter ( Fig. 2c ) and chromatin immunoprecipitation (ChIP) analyses confirmed significant KLF15 occupancy at multiple consensus binding sites (CACCC or G/C-rich elements) within the endogenous Fgf15 promoter ( Fig. 2d ; the KChip2 promoter serves as positive control [18] ). In addition, Fgf15 was strongly induced in the Klf15 −/− ileum (and modestly in jejunum) as assessed by quantative PCR (qPCR) analysis ( Fig. 2e ) and confirmed by ISH ( Fig. 2a , far right panel). Finally, given that KLF15 is a circadian factor, we assessed Klf15 and Fgf15 expression across a 24-h cycle. As shown in Fig. 2f–i , Klf15 and Fgf15 mRNA and protein expressions (by western blot or plasma enzyme-linked immunosorbent assay (ELISA)) both oscillated in ileal tissues and blood. Importantly, in the absence of Klf15 , ileal Fgf15 mRNA expression and serum FGF15 levels were increased at multiple time points across a 24-h cycle. Collectively, these data identify KLF15 as a direct negative regulator of Fgf15 . 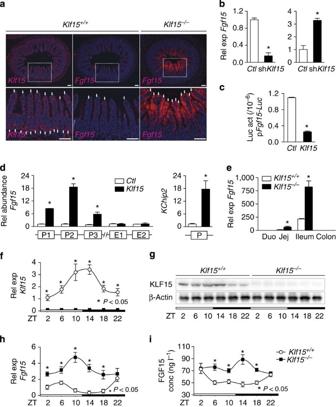Figure 2: Ileal KLF15 regulates circadian FGF15 production to control BA synthesis. (a)In situhybridization analysis ofKlf15andFgf15expression inKlf15+/+andKlf15−/−mouse ileum. White arrows indicateKlf15orFgf15mRNA signal. (b) Effects of adenoviral overexpression and shRNA knockdown ofKlf15onFgf15mRNA expression in primary mouse small intestinal epithelial cells. Primary small intestinal epithelial cells were infected with control virus (Ctl), adKlf15, or shKlf15as indicated. (c)Fgf15-Lucreporter assay in Caco2 cells following heterologous overexpression ofFlag-Klf15(Klf15) orpc-DNA3.1(control,Ctl). (d) ChIP analysis of KLF15 (Flag-Klf15) binding to designate regions of theFgf15and the Kv channel-interacting protein 2 (KChip2) promoters in the mouse colon cell line CT26. The relative binding abundance (Rel abundance) was normalized to IgG. (e)Fgf15mRNA expression inKlf15+/+versusKlf15−/−mouse intestine segments: Duo, Jej, ileum and colon (n=8). (f) Circadian rhythm ofKlf15mRNA expression inKlf15+/+mouse ileum (P<0.01) was abolished inKlf15−/−mouse ileum (n=5 per time point). (g) Immunoblot of circadian KLF15 protein expression in the ileum (representative of three experiments). IlealFgf15mRNA expression (h) and blood FGF15 protein concentrations (Conc) (i) exhibit circadian variations inKlf15+/+mice (P<0.01) but the rhythms inKlf15−/−mice were lost with increased expression at indicated time points (n=5). Data represent mean±s.e.m. Statistical significance of circadian rhythm for each genotype was analysed using analysis of variance followed by Bonferroni post-test. Statistical significance between the two individual groups was assessed using Student’st-test. * indicatesP<0.05, compared with control (Ctl), orKlf15+/+mice. Scale bars, 100 μm (a). Figure 2: Ileal KLF15 regulates circadian FGF15 production to control BA synthesis. ( a ) In situ hybridization analysis of Klf15 and Fgf15 expression in Klf15 +/+ and Klf15 −/− mouse ileum. White arrows indicate Klf15 or Fgf15 mRNA signal. ( b ) Effects of adenoviral overexpression and shRNA knockdown of Klf15 on Fgf15 mRNA expression in primary mouse small intestinal epithelial cells. Primary small intestinal epithelial cells were infected with control virus ( Ctl ), ad Klf15 , or sh Klf15 as indicated. ( c ) Fgf15-Luc reporter assay in Caco2 cells following heterologous overexpression of Flag-Klf15 ( Klf15 ) or pc-DNA3.1 (control, Ctl ). ( d ) ChIP analysis of KLF15 ( Flag-Klf15 ) binding to designate regions of the Fgf15 and the Kv channel-interacting protein 2 ( KChip2 ) promoters in the mouse colon cell line CT26. The relative binding abundance (Rel abundance) was normalized to IgG. ( e ) Fgf15 mRNA expression in Klf15 +/+ versus Klf15 −/− mouse intestine segments: Duo, Jej, ileum and colon ( n =8). ( f ) Circadian rhythm of Klf15 mRNA expression in Klf15 +/+ mouse ileum ( P <0.01) was abolished in Klf15 −/− mouse ileum ( n =5 per time point). ( g ) Immunoblot of circadian KLF15 protein expression in the ileum (representative of three experiments). Ileal Fgf15 mRNA expression ( h ) and blood FGF15 protein concentrations (Conc) ( i ) exhibit circadian variations in Klf15 +/+ mice ( P <0.01) but the rhythms in Klf15 −/− mice were lost with increased expression at indicated time points ( n =5). Data represent mean±s.e.m. Statistical significance of circadian rhythm for each genotype was analysed using analysis of variance followed by Bonferroni post-test. Statistical significance between the two individual groups was assessed using Student’s t- test. * indicates P <0.05, compared with control ( Ctl ), or Klf15 +/+ mice. Scale bars, 100 μm ( a ). Full size image Ileectomy restores BA synthesis in Klf15 −/− mice The above data are consistent with a model in which ileal KLF15 controls Cyp7a1 expression in the liver by regulating ileal Fgf15 . Resection of ileum restored plasma FGF15 levels, Cyp7a1 mRNA expression and BA amounts in Klf15 −/− mice to levels comparable to Klf15 +/+ mice ( Fig. 3a–d ). Similar results were found after both ileal and jejunal resection ( Supplementary Fig.5a,b ). As FGF15 binding to its receptor FGFR4 is critical for inhibition of Cyp7a1 and BA production, we next sought to determine whether FGFR4 was required for KLF15-mediated downregulation of Fgf15 . Tail-vein injection of adenoviral Fgfr4 short hairpin RNA (shRNA) efficiently reduced mRNA expression by ∼ 90% ( Fig. 3e ). Critically, the reduced expression of Cyp7a1 in Klf15 −/− mice was completely abrogated to levels comparable to those observed in Klf15 +/+ mice following Fgfr4 depletion. Collectively, the results of Figs 2 and 3 suggest that KLF15-dependent regulation of ileal Fgf15 is critical for Cyp7a1 expression and BA synthesis in the liver. 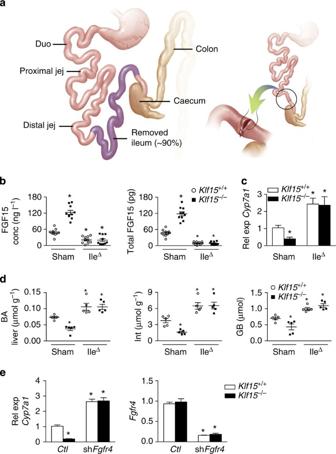Figure 3: Ileectomy and knockdown of hepaticFgfr4restoreCyp7a1expression and BA synthesis inKlf15−/−mice. (a) Schematic picture before and after ileectomy (IleΔ). Approximately 90% of the ileum was resected. (b) FGF15 protein concentration (left) and total amount (right) in blood fromKlf15+/+andKlf15−/−mice at ZT14 after sham or IleΔsurgery (n=10). (c) The mRNA levels of hepaticCyp7a1inKlf15+/+andKlf15−/−mice at ZT14 after sham or IleΔ(n=5). (d) BA amount in liver, intestine (Int) and GB inKlf15+/+versusKlf15−/−, sham versus IleΔmice (n=5). (e) mRNA expression of the liverCyp7a1andFgfr4inKlf15+/+andKlf15−/−mice infected with adenoviral shRNA control (Ctl) or shFgfr4(n=5). Statistical significance between the two individual groups was assessed using Student’st-test. Normal distribution was assumed. * indicatesP<0.05, compared withKlf15+/+mice with sham surgery or infected withCtl. Figure 3: Ileectomy and knockdown of hepatic Fgfr4 restore Cyp7a1 expression and BA synthesis in Klf15 −/− mice. ( a ) Schematic picture before and after ileectomy (Ile Δ ). Approximately 90% of the ileum was resected. ( b ) FGF15 protein concentration (left) and total amount (right) in blood from Klf15 +/+ and Klf15 −/− mice at ZT14 after sham or Ile Δ surgery ( n =10). ( c ) The mRNA levels of hepatic Cyp7a1 in Klf15 +/+ and Klf15 −/− mice at ZT14 after sham or Ile Δ ( n =5). ( d ) BA amount in liver, intestine (Int) and GB in Klf15 +/+ versus Klf15 −/− , sham versus Ile Δ mice ( n =5). ( e ) mRNA expression of the liver Cyp7a1 and Fgfr4 in Klf15 +/+ and Klf15 −/− mice infected with adenoviral shRNA control ( Ctl ) or sh Fgfr4 ( n =5). Statistical significance between the two individual groups was assessed using Student’s t -test. Normal distribution was assumed. * indicates P <0.05, compared with Klf15 +/+ mice with sham surgery or infected with Ctl . Full size image KLF15 regulates FGF15 and BA synthesis in a BA-independent manner Recent literature suggests that BA-dependent activation of FXR in epithelial cells of the distal ileum leads to Fgf15 production. However, our mechanistic data raises the possibility that KLF15 may directly regulate Fgf15 . If this hypothesis is correct, then the effect of Klf15 deficiency on Fgf15 and Cyp7a1 expression and BA production should be preserved in the absence of BA. To address this hypothesis, we employed a bile duct catheterization (BDC) model in mice that captures BAs before they can enter the small bowel ( Fig. 4a ; Supplementary Fig. 6a ). This approach also allows for quantification of BA production while avoiding BA-induced hepatic toxicity that may occur with ligation of the bile duct. Importantly, the oscillation of ileal Fgf15 , ileal Klf15 and hepatic Cyp7a1 at ZT2 and ZT14 was maintained after BDC ( Supplementary Fig. 6b,c ). Further, the expected effect of Klf15 deficiency on Fgf15 / Cyp7a1 expression was present after sham surgery ( Fig. 4b,c ). Importantly, following BDC, the expression of ileal Fgf15 in Klf15 −/− animals remained significantly higher ( Fig. 4b ), while hepatic Cyp7a1 ( Fig. 4c ), BA volume ( Fig. 4d,e ) and total BA amount ( Fig. 4f ) were lower. These data demonstrate that KLF15 regulation of Fgf15 occurs in a BA-independent manner. 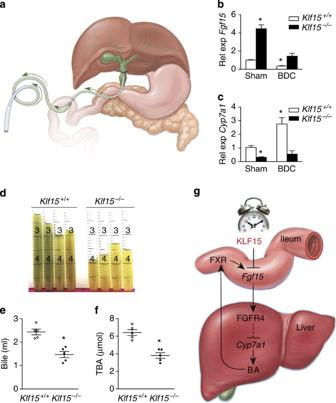Figure 4: KLF15 inhibitsFgf15and induces BA synthesis in a BA-independent manner. (a) Schematic representation of bile duct catheterization (BDC). mRNA expression of intestinalFgf15(b)and liverCyp7a1(c)inKlf15+/+andKlf15−/−mice at ZT14 after sham or BDC surgery (n=5). (d) Bile collected fromKlf15+/+andKlf15−/−mice 24 h after BDC surgery (one mouse bile/tube). (e) Bile total volume inKlf15+/+andKlf15−/−mice 24 h after BDC surgery. (f) Total BA (TBA) amount in collectedKlf15+/+andKlf15−/−mouse bile (n=5 per group). (g) Schematic model of KLF15 regulation of mouseCyp7a1gene expression and BA synthesis. Statistical significance between the two individual groups was assessed using Student’st-test. Normal distribution was assumed. * indicatesP<0.05, compared with sham orKlf15+/+mice. Figure 4: KLF15 inhibits Fgf15 and induces BA synthesis in a BA-independent manner. ( a ) Schematic representation of bile duct catheterization (BDC). mRNA expression of intestinal Fgf15 (b) and liver Cyp7a1 (c) in Klf15 +/+ and Klf15 −/− mice at ZT14 after sham or BDC surgery ( n =5). ( d ) Bile collected from Klf15 +/+ and Klf15 −/− mice 24 h after BDC surgery (one mouse bile/tube). ( e ) Bile total volume in Klf15 +/+ and Klf15 −/− mice 24 h after BDC surgery. ( f ) Total BA (TBA) amount in collected Klf15 +/+ and Klf15 −/− mouse bile ( n =5 per group). ( g ) Schematic model of KLF15 regulation of mouse Cyp7a1 gene expression and BA synthesis. Statistical significance between the two individual groups was assessed using Student’s t -test. Normal distribution was assumed. * indicates P <0.05, compared with sham or Klf15 +/+ mice. Full size image The circadian nature of BA synthesis has been known for >50 years [19] . Given the importance of BAs in nutrient availability and metabolic homeostasis, the molecular basis for this oscillatory behaviour has been the subject of great interest. The present study identifies a novel KLF15- Fgf15 pathway that regulates this process ( Fig. 4g ). Specifically, we establish KLF15 as a novel regulator of BA synthesis, show that KLF15 exacts this effect by repressing Fgf15 , and demonstrate that the circadian regulation of Fgf15 is independent of BA stimulation. These findings, in the context of elegant published work [9] , suggest a dual mechanism underlying Fgf15 production: cyclical expression of ileal KLF15 in addition to the well-established pathway that involves BA-dependent activation of the nuclear receptor FXR. However, our work does not exclude the possibility that additional mechanisms may be operative by which KLF15 may affect Fgf15 and consequently BA production. Indeed, we observed that KLF15 could repress Fgf15 expression induced by a synthetic FXR agonist ( Supplementary Fig. 4 ) indicating that, in principle, additional mechanisms may contribute. This is an intriguing question worthy of further study. The KLF15- Fgf15 pathway reported here may have important implications for the metabolism beyond the regulation of BA. FGF15 has been characterized as a ‘long-acting insulin’ with effects on glucose homeostasis following feeding [20] . Studies over the past decade have implicated KLF15 in regulation of gluconeogenesis in the context of nutrient deprivation [17] raising the possibility that the antagonistic relationship between KLF15 and FGF15 may have important implications for glucose metabolism in a number of physiologic states. Finally, the fact that KLF15 has been shown to regulate glucose [16] , lipid [21] and amino-acid [16] metabolism coupled with the current insights related to nutrient availability suggest that KLF15 serves as a major node for systemic metabolic homeostasis. Mice All animal studies were carried out with permission, and in accordance with animal care guidelines from the Institutional Animal Care Use Committee at Case Western Reserve University and at collaborating facilities. Generation of systemic Klf15 -null ( Klf15 −/− ) mice has been previously described [11] . Klf15 −/− mice were backcrossed onto a C57BL/6J background for over 10 generations. Age-matched wild-type ( Klf15 +/+ ) and Klf15 −/− male mice on C57BL/6J background (Jackson Laboratory, Bar Harbor, ME, USA) were bred in our facility and used for circadian and other studies such as ileectomy and BDC. Mice were housed under light–dark (12 h/12 h) conditions: lights on at 06:00 (ZT0) and lights off at 18:00 (ZT12). Mice had free access to standard chow and water. Liver-specific Klf15 -knockout mice were generated by breeding Alb-Cre mice and floxed- Klf15 mice to generate Alb-Cre /floxed- Klf15 (Li-KO) mice. For circadian studies, 8–12-week-old male mice were killed with isoflurane every 4 h for 24 h. Blood and tissues were harvested for mRNA, protein and other assays. Cell culture and reagents Hepa1-6 (ATCC, Manassas, VA, USA) hepatocytes were maintained in DMEM (Invitrogen/Life Technologies, Grand Island, NY, USA) supplemented with 10% foetal bovine serum (FBS) and 1% penicillin/streptomycin. Murine CT26 colonic cells (ATCC) were maintained in RPMI media (Invitrogen) supplemented with 20% FBS and 1% penicillin/streptomycin. Human Caco2 colonic cells (ATCC) were maintained in EMEM (ATCC) supplemented with 20% FBS and 1% penicillin/streptomycin. Primary mouse small intestine epithelial cells were purchased from Cell Biologics Inc. (Chicago, IL, USA) and cultured in epithelial cell medium containing 0.1% epidermal growth factor, 0.1% insulin-transferrin sodium selenite, 0.1% hydrocortisone, 5% FBS, 1% L-glutamine and a 1% antibiotic-antimycotic solution on gelatin (Sigma-Aldrich, St Louis, MO, USA)-coated plates. GW4064 was purchased from Sigma-Aldrich. Isolation of primary mouse hepatocytes Mice (8-week-old male) were anaesthetized by ketamine/xylazine. All media were purchased from Gibco/Life Technologies. Following dissection to expose the inferior vena cava (IVC), a catheter was inserted into the IVC, tightened by a suture and then connected to the perfusion pump with liver perfusion media. The thorax was quickly opened to clamp off the IVC above the diaphragm and the portal vein was cut. The perfusion was continued at 8 ml min −1 for 5 min. The liver was then perfused with collagenase I containing liver digestion media with at 8 ml min −1 for 6 min. Digested liver was minced and shaken vigorously to release hepatocytes in cold hepatocyte wash media. The suspension was filtered through a 70-μm cell strainer and centrifuged at 50 g for 3 min. Hepatocytes were resuspended by William's E media, seeded in collagen I-coated plates and cultured in HepatoZYME serum-free media. RNA purification, reverse transcription (RT) and RT–qPCR RNA was extracted from mouse tissues or cells using column-based Aurum total RNA fatty and fibrous tissue kit following the manufacturer’s instructions (Bio-Rad, Hercules, CA, USA). Purified RNA (1 μg) was subject to reverse transcription using iScript Reverse Transcription Supermix for RT–qPCR kit (Bio-Rad). Resulting complementary DNA (cDNA) was analysed by RT–qPCR. Briefly, 2 μl of cDNA and 1 μl of each primer were mixed with TaqMan qPCR Master Mix (Applied Biosystems/Life Technologies). Reactions were performed in 384-well format using an ABI One Plus instrument (Applied Biosystems). Relative mRNA levels were calculated using the comparative Ct method normalized to 18S . All the primers and probes were designed using Primer Express Software (Roche, Indianapolis, IN, USA) for Cyp7a1 , Cyp7b1 , Cyp27a1 , Fxr , Shp , Klf15 , Fgf15 , liver receptor homologue-1 ( Lrh1/Nr5a2 ), hepatocyte nuclear factor 4a ( Hnf4a/Nr2a1 ), liver X receptor ( Lxr/Nr1h3 ), Fgfr4 and 18S ( Supplementary Table 1 ). Molecular biology Adenoviral overexpression studies in mouse primary small intestinal epithelial cells were performed using an adenoviral construct carrying the mouse Klf15 gene (ad Klf15 ) or empty control virus ( Ctl ) as previously described [17] . Knockdown of Klf15 was achieved using a Klf15 shRNA construct (sh Klf15 ) or empty control virus shRNA ( Ctl ) as previously described [21] . To clone the Fgf15 promoter reporter construct, mouse genomic DNA was first isolated from mouse liver using a genomic DNA isolation kit (Qiagen, Germantown, MD, USA). The mouse Fgf15 promoter from −2,952 to −60 (2,893 bp) was amplified from genomic DNA by PCR (CloneAmp HiFi PCR Premix, Clontech, Mountain View, CA, USA) and inserted into a pGL3 luciferase reporter vector using restriction sites digested by Nhe I and Xho I (New England Biolabs Inc., Ipswich, MA, USA). The sequences of primers for Fgf15 promoter: forward, 5′-gatcGCTAGCGCTGTCTTCAGACACAC-3′ and reverse, 5′-GCTCGGGCCACCGCACCTCGAGgatc-3′. ISH of Fgf15 expression in the mouse ileum was carried out using a truncated clone of Fgf15 cDNA as an ISH probe, which has been previously described [22] . RNA extraction from Klf15 −/− mouse ileum and RT were described above. The cDNA was subjected to PCR to amplify the Fgf15 cDNA fragment. The sequences of primers for Fgf15 cDNA: forward, 5′-CCAGTTGCTTTGTGGGTTGTGCCT-3′ and reverse, 5′- AAGTTCACGGGACCTTGGGGTTTTC-3′. ISH of Klf15 expression in the mouse ileum was carried out using a truncated clone of Klf15 cDNA as an ISH probe. RNA was extracted from Klf15 +/+ mouse ileum and RT. The cDNA was subjected to PCR to amplify the Klf15 cDNA fragment. The sequences of primers for Klf15 cDNA: forward, 5′-TGTGAAGCCGTACCAGTGTC-3′ and reverse, 5′-CCTGTCAAAACAAGCTAGTTCAA-3′. The amplified cDNA fragments were inserted into the pCR2.1-TOPO vector (Invitrogen). Knockdown of Fgfr4 in vivo Knockdown of liver Fgfr4 was achieved using commercial Fgfr4 shRNA construct (sh Fgfr4 ) or empty control virus ( Ctl ) provided by Vector Lab (Philadelphia, PA, USA). Mice (8–12-week-old male) were used for the tail-vein injection with shFgfr4 or control constructs (10 9 plaque-forming unit per mouse). The mice were killed 3 days after infection for the biochemical and molecular studies. Western blotting assay Liver samples were homogenized in modified RIPA buffer containing 50 mM Tris, 150 mM NaCl, 1 mM EDTA, 1% Triton X-100, 0.5% sodium deoxycholate and 1% SDS supplemented with protease and phosphatase inhibitors (Roche). CYP7A1 (Catalog #: sc25536, 200 μg ml −1 , 1:500 dilution), CYP7B1 (Catalog #: sc26087, 200 μg ml −1 , 1:500 dilution) and β-actin (Catalog #: sc47778, 200 μg ml −1 , 1:1,000 dilution) antibodies were purchased from Santa Cruz and KLF15 (Catalog #: ab2647, 0.5 mg ml −1 , 1:1,000 dilution) antibody was from Abcam (Cambridge, MA, USA) for immunoblot analyses. Immunoblot signals were quantified using ImageJ (ImageJ 1.48v, NIH). Full-length images of immunoblots are shown in Supplementary Figures 7–8 . Tissue harvest and biochemical analysis of BAs BA extraction was performed as previously descrived [23] , [24] . BAs in the liver, intestine and GB were extracted with 95% ethanol once overnight. Tissues were then extracted by 80% ethanol once for 2 h, and further extracted by chloroform/methanol (2:1) once for 2 h at 50 °C. BAs were determined using a bile acid assay kit (Genzyme Diagnostic, Framingham, MA, USA). Ileectomy or resection of ileum and jejunum Mice (8–12-week-old male) were used for surgery. Mice were anaesthetized with isoflurane (1–2%), and placed on a temperature-controlled small animal surgical table to maintain body temperature during surgery. A midline incision was made in the abdomen to expose the intestine. The segment of ∼ 90% ileum or ileum and jejunum was cut-off, and warm saline and antibiotics were used to wash the cut ends. Both cut ends were further trimmed off about 2 mm, and then anastomosed with 7-0 suture. The surgery area was washed with warm saline and antibiotics. The incision of abdomen was closed with 5-0 suture. Blood and tissues were harvested for molecular and biochemical analyses 24 h after surgery. Bile duct catheterization (BDC) Mice (8–12-week-old male) were used for sham or BDC. Mice were anaesthetized with isoflurane (1–2%), and placed on a temperature-controlled small animal surgical table. A midline incision in the abdomen was made to expose the bile duct. The common bile duct was catheterized at the upper margin of the pancreas using a segment of micro-miniature tubing (SUBL-190, Braintree Scientific Inc., Braintree, MA, USA) connected to a silicone tubing (SIL-025, Braintree Scientific Inc.). The incision of subcutaneous membrane was closed with 5-0 sutures. The end of the tubing was left out of the abdomen, and connected to another bile collection tubing (0.062 inch ID, Helix Medical, LLC, Carpentaria, CA, USA). The collection tubing was rolled and placed subcutaneously. The surgery area was washed with warm saline and antibiotics solution. The incision of abdomen skin was closed with 5-0 sutures. Bile was harvested from the tube twice at ZT2 and ZT14 after the BDC. After the second collection, tissues and blood were harvested for further analyses. ELISA assay Mouse FGF15 ELISA kit (Catalog #: MBS161951) was purchased from MyBioSource (San Diego, CA, USA). Mouse blood was collected by heparin rinsed syringe, stored in EDTA-coated tubes and spun at 300 g for 20 min. Plasma or FGF15 standards (40 μl per each) were added to the ELISA plate, which had been pre-coated with FGF15 monoclonal antibody. Anti-FGF15 antibody labelled with biotin was added and incubated with streptavidin-horseradish peroxidase to form immune complex. The plate was incubated for 1 h at 37 °C without exposure to the light. Nonspecific binding was washed away, and substrates A and B were added to the wells. The absorbance was read at 450 nm. The absorbance and the concentration of mouse FGF15 were positively correlated. A background of ∼ 30 ng l −1 was observed when Fgf15 -knockout mouse plasma was used for FGF15 measurement. Total blood volume per mouse was multiplied with the FGF15 concentration to generate total circulating FGF15 amount. Reporter assay Mouse Cyp7a1-Luc reporter construct (1 kb), and human LXR , LRH1 , HNF4A and RXR expression plasmids were generously provided by Dr John Chiang at Northeast Ohio Medical University (Rootstown, OH, USA). Hepa1-6 cells were transfected with Cyp7a1-Luc , and LXR , LRH1 , HNF4A , RXR , Flag-Klf15 and/or pcDNA3.1 ( Control , Ctl) constructs using X-treme GENE HP DNA transfection reagent (Roche). Caco2 cells were transfected with Fgf15-Luc reporter constructs and Flag-Klf15 plasmids. Luciferase activity in transfected cells was measured using a luciferase reporter assay system (Promega, Madison, WI, USA). Luciferase activity was normalized to total cell protein concentration (BCA kit, Pierce Biotechnology/Thermo Scientific, Rockford, IL, USA). ChIP assay Mouse colon cell line CT26 cells were subjected to the ChIP analysis using a commercial ChIP assay kit (Millipore, Billerica, MA, USA). Briefly, cells were cultured to ∼ 70% confluence and then transfected with Flag-Klf15 or pcDNA3.1 constructs for 24 h. Cells were fixed with fresh 1% formaldehyde at room temperature for 10 min, and then neutralized by glycine. Cells were washed by PBS, and collected and pelleted at 800 g for 5 min. Cells were lysed with cell lysis buffer to release nuclei, which were then lysed with nucleus lysis buffer. The nuclear lysates were sonicated on ice with the sonicator (Diagenode, Denville, NJ, USA) with 30% output for 6 × 10 s. The sonicated chromatin was immunoprecipitated using anti-Flag (Sigma) or non-immune IgG (Epigetek Group Inc., Farmingdale, NY, USA) and bound to Dynabeads. The yielded chromatin fragments were analysed by ChIP primers using SYBR GreenERTM PCR Master Mix (Roche). Five pairs of primers were used for ChIP of the Fgf15 promoter and expression regions ( Supplementary Table 2 ). The relative abundance was normalized to abundance of IgG as previously described [25] . In situ hybridization Samples were fixed overnight with 4% paraformaldehyde and dehydrated through an ethanol series. Samples were then paraffin embedded and sectioned. Radioactive ISHs were performed using previously described protocols [26] . Probes for Klf15 and Fgf15 were described in Molecular Biology section above. Brightness and contrast of ISH images were adjusted identically in all control and mutant images using Adobe Photoshop. Lipid infusion and absorption The method used has been described in detail by Tso and Simmonds [27] . In brief, mice were infused with a lipid diet with labelled [ 3 H] triolein (TG) and [ 14 C] cholesterol into the duodenum at 0.3 ml h −1 for 6 h. At the end of infusion, the animals were anaesthesized and the small intestine (from duodenum to ileum) was cut into four equal segments referred to as L1–L4. L1 contains luminal content from proximal segment of small intestine, duodenum; L2 and L3 contain luminal content from jejunum; L4 contains luminal content from ileum. Luminal lipids were harvested by washing each intestinal segment with 0.5% sodium taurocholate in saline and radioactivity of luminal contents measured by liquid scintillation counting. The presence of higher amounts of labelled TG or cholesterol in the duodenal lumen indicated reduced lipid absorption. Statistical analysis All data were presented as mean±s.e.m. ( n as indicated in the figure legends). The statistical difference between the two individual groups was assessed using Student’s t -test. For circadian mouse studies, the GraphPad software Prism (Prism 5, GraphPad Software Inc.) was used. The statistical significance between time points to assess the rhythmicity was performed using one-way analysis of variance. Circadian differences between Klf15 +/+ and Klf15 −/− mice were assessed using two-way analysis of variance followed by Bonferroni post-test. Normal distribution was assumed for all experimental groups. P <0.05 was considered statistically significant. How to cite this article: Han, S. et al . Circadian control of bile acid synthesis by a KLF15- Fgf15 axis. Nat. Commun. 6:7231 doi: 10.1038/ncomms8231 (2015).